A chemical genetic screen inMycobacterium tuberculosisidentifies carbon-source-dependent growth inhibitors devoid ofin vivoefficacy Candidate antibacterials are usually identified on the basis of their in vitro activity. However, the apparent inhibitory activity of new leads can be misleading because most culture media do not reproduce an environment relevant to infection in vivo . In this study, while screening for novel anti-tuberculars, we uncovered how carbon metabolism can affect antimicrobial activity. Novel pyrimidine–imidazoles (PIs) were identified in a whole-cell screen against Mycobacterium tuberculosis . Lead optimization generated in vitro potent derivatives with desirable pharmacokinetic properties, yet without in vivo efficacy. Mechanism of action studies linked the PI activity to glycerol metabolism, which is not relevant for M. tuberculosis during infection. PIs induced self-poisoning of M. tuberculosis by promoting the accumulation of glycerol phosphate and rapid ATP depletion. This study underlines the importance of understanding central bacterial metabolism in vivo and of developing predictive in vitro culture conditions as a prerequisite for the rational discovery of new antibiotics. The field of anti-tuberculosis drug discovery culminated in the 1960s with the incorporation of rifampicin and pyrazinamide in the tuberculosis drug regimen. The use of these two antimicrobials, in combination with isoniazid, ethambutol and/or streptomycin, represents a landmark in the treatment of human tuberculosis and resulted in the implementation of short-course chemotherapy (SCC), reducing the time of treatment from 18 to 6 months [1] , [2] , [3] . Short-course chemotherapy contributed towards controlling tuberculosis burden for the next 20 years. Nevertheless, tuberculosis cases started to rise again in the 1990s under the pressure of the HIV pandemic and the emergence of multidrug-resistant (MDR) and extremely drug-resistant (XDR) tuberculosis strains. MDR strains are resistant to at least isoniazid (INH) and rifampicin (RIF), whereas XDR strains are MDR isolates that are additionally resistant to fluoroquinolones and to one of the three injectable drugs capreomycin, amikacin and kanamycin. The emergence and dissemination of MDR and XDR isolates, estimated to account for more than 400,000 new cases per year, impart new challenges in tuberculosis control [4] . Indeed, current treatment of drug-resistant tuberculosis requires 18–36 months and is associated with an unacceptable rate of treatment failure and relapse. Consequently, developing new compounds active against MDR and XDR tuberculosis constitutes a main objective in anti-tuberculosis drug discovery. In addition, new antimycobacterial agents should ideally contribute to shorten tuberculosis treatment to 2 months or less [5] , [6] . Few promising drug candidates fulfilling these criteria have been discovered in recent years [7] , [8] , [9] . Of particular interest is TMC207, which has been shown to be highly active in proof-of-concept trials, and shows the potential to shorten the duration of therapy [10] . Nonetheless, given the number of tuberculosis cases and the rate of emergence of drug resistance, more compounds are clearly needed to combat and have a significant impact on the control and spread of tuberculosis. Target- and cell-based screens are the two main approaches used to identify new antibacterials. With the recent development of miniaturized high-throughput screening technologies and methods such as fragment-based screening [11] , target-based screens seem very attractive as they allow for the rational discovery and optimization of new antibacterial leads. However, these approaches have failed to meet expectations and have proved to be unsuccessful in the identification of novel antimicrobials in general [12] . Reasons for this lack of success are not entirely clear but may be partially attributed to the lack of a validated target, and the difficulty in predicting the biological effect on target inhibition on the whole bacterium [13] . In contrast, all existing antibacterials on the market and/or in clinical development have been identified through cell-based screening methods. The major advantage of cellular screens lies in the possibility of identifying compounds with a complex and pleiotropic mode of action resulting in cellular death [13] , [14] . Such a category of compounds cannot be rationally obtained from a classical target-based screen. A common issue inherent to target- and cell-based assays is the limited predictive value of the in vitro culture conditions used to test novel compounds. This limitation is not restricted to tuberculosis drug development, as recently illustrated while validating the type II fatty acid synthesis (FASII) pathway as a drug target against Gram-positive bacteria [15] . The FASII pathway was proposed to be an attractive target based on genetic essentiality in vitro and on the discovery of promising lead candidates [16] , [17] , [18] . However, Gram-positive bacteria were shown to acquire complex host-derived lipids in vivo , bypassing the essentiality of the FASII system described in vitro [15] , thereby rendering the FASII pathway futile as a drug target. This observation highlights the need to develop predictive in vitro culture conditions for screening and testing new antibiotics. Most culture media currently used for anti-tubercular compound testing were all developed empirically several decades ago for optimal propagation of the bacilli in vitro [19] , [20] , [21] , [22] . These media were not optimized for drug screening, nor were they meant to reproduce the environmental conditions encountered in the infected host. This study underlines the largely overlooked yet crucial importance of culture conditions and its impact on the disconnect between in vitro potency and in vivo efficacy in antibacterial drug discovery. Here, a new class of compounds active against Mycobacterium tuberculosis was identified through a whole-cell screen. Despite excellent in vitro activity and desirable pharmacological properties, the optimized compounds were found to be inactive in a tuberculosis mouse model. The disconnect between in vitro activity and in vivo efficacy was explained by a major difference in carbon metabolism between bacteria replicating in standard tuberculosis broth medium as compared with infected lungs. Identification of a new class of anti-tubercular compounds A cellular screen was developed to identify mycobacterial growth inhibitors. The screen was carried out against M. bovis BCG using intracellular ATP content as a surrogate marker of bacillary growth. Compound hits with confirmed activity against M. tuberculosis were chemically clustered to identify any emerging structure–activity relationship. Our attention was drawn to a cluster of pyrimidine–imidazole (PI) compounds comprising five compounds with an MIC 50 ranging from 0.11 to >20 μM ( Supplementary Table S1 ). The compounds were bactericidal and the cytotoxic profile was within an acceptable range ( Supplementary Table S1 ). Therefore, a lead optimization programme was initiated with the goal of achieving desirable in vivo PK properties while retaining the potent anti-tubercular activity. Optimized PI compounds are not efficacious in vivo A total of 324 derivatives were synthesized. 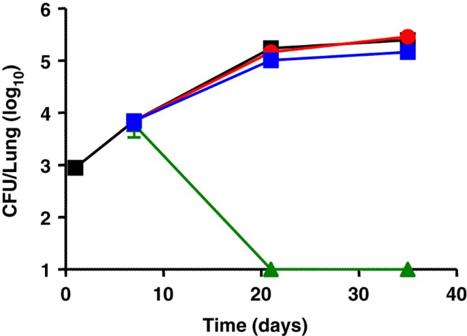Figure 1:In vivoactivity of compound3in the mouse model. Balb/C mice were infected intranasally with∼103M. tuberculosis H37Rv. Drug treatment was initiated 1 week after infection and was administered orally for 28 days daily at 25 mg kg−1(red circles) and 100 mg kg−1(blue diamonds). Bacterial loads were determined after 14 and 28 days of drug treatment and compared with the control group (HPβCD formulation alone, black squares). Isoniazid (green triangles, 25 mg kg−1) was used as a positive control. Compounds 1 , 2 and 3 ( Table 1 ) were selected for efficacy testing in the mouse model. 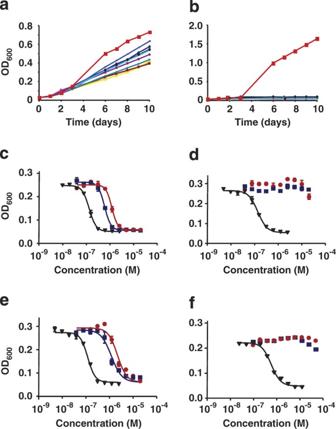Figure 2: Glycerol dissimilation is required for the anti-tubercular activity of the PI compounds. M. tuberculosisH37Rv (red squares) and spontaneous mutants resistant to2(clones 1–9, other symbols) were incubated in a medium containing a complex mixture of carbon sources (7H9 medium,a), or in a medium containing glycerol as the sole carbon source (Sauton medium,b). Growth was monitored by following the OD600over time. The MIC50of1(red circles) and2(blue squares) was tested against the parental H37Rv strain (c,f), H37Rv ΔglpKstrain (d) and H37Rv ΔglpKpMV306-glpK(e) in the presence (c–e) or absence (f) of glycerol. Streptomycin (black triangles) was used as a reference compound. In vivo PK studies in the mouse revealed oral bioavailability ranging between 50 and 100% ( Table 2 ). Following a dose of 25 mg kg −1 , lung levels were above the minimum inhibitory concentration (MIC) for 30–100% of the dosing interval ( Table 2 ). Additional PK studies at 100 mg kg −1 showed that exposure of 3 was proportional to dose, providing plasma and lung levels were above the MIC for the entire dosing interval ( Table 2 ). Pharmacokinetic/pharmacodynamic (PK/PD) indices corrected for protein binding were favourable, with 3 at 100 mg kg −1 showing PK/PD indices similar to those of isoniazid ( Table 2 ). However, when tested in the tuberculosis mouse model at 25 and 100 mg kg −1 , all three compounds were found to be ineffective in reducing lung bacterial loads, despite 28-day courses of daily dosing ( Fig. 1 ; data not shown). Table 1 Structure and biological activity of the PI compounds. Full size table Table 2 PK/PD parameters of 1–3. Full size table Figure 1: In vivo activity of compound 3 in the mouse model. Balb/C mice were infected intranasally with ∼ 10 3 M. tuberculosi s H37Rv. Drug treatment was initiated 1 week after infection and was administered orally for 28 days daily at 25 mg kg −1 (red circles) and 100 mg kg −1 (blue diamonds). Bacterial loads were determined after 14 and 28 days of drug treatment and compared with the control group (HPβCD formulation alone, black squares). Isoniazid (green triangles, 25 mg kg −1 ) was used as a positive control. Full size image These results underline how anti-tubercular compounds with good in vitro activity and good PK/PD properties can still be without in vivo activity. PI compounds are inactive in the absence of glycerol In an attempt to understand the disconnect between in vitro activity and in vivo efficacy of the PI compounds, M. tuberculosis spontaneous mutants resistant to 2 were isolated. The clones obtained were highly resistant to the PI compounds with MIC 50 values greater than 20 μM. In addition, the spontaneous mutants resistant to 2 were cross-resistant to 1 and 3 , with MIC 50 greater than 20 μM. Full-genome sequencing of four independently isolated resistant mutants revealed a single polymorphism in glpk , which encodes for glycerol kinase (GlpK, Rv3696c), the first committing enzyme for glycerol metabolism in most bacteria. One of the four clones showed a single-nucleotide polymorphism at codon 187 ( 187 GGG> 187 G T G), whereas the other three clones harboured a frameshift mutation due to the insertion of a guanine in codon 191 ( 191 GGT> 191 GG G T). Mutation 191 GGT> 191 GG G T was identified by sequencing in five additional spontaneous-resistant mutants. Interestingly, the same frameshift mutation is naturally found in some M. bovis strains, a species unable to metabolize glycerol [23] . M. bovis BCG, the mycobacterial species used for the whole-cell screen, can metabolize glycerol and has no frameshift mutation in glpK [23] . Consistently, none of the spontaneous-resistant mutants was able to multiply in the presence of glycerol as the sole carbon source ( Fig. 2a,b ). Figure 2: Glycerol dissimilation is required for the anti-tubercular activity of the PI compounds. M. tuberculosis H37Rv (red squares) and spontaneous mutants resistant to 2 (clones 1–9, other symbols) were incubated in a medium containing a complex mixture of carbon sources (7H9 medium, a ), or in a medium containing glycerol as the sole carbon source (Sauton medium, b ). Growth was monitored by following the OD 600 over time. The MIC 50 of 1 (red circles) and 2 (blue squares) was tested against the parental H37Rv strain ( c , f ), H37Rv Δ glpK strain ( d ) and H37Rv Δ glpK pMV306- glpK ( e ) in the presence ( c – e ) or absence ( f ) of glycerol. Streptomycin (black triangles) was used as a reference compound. Full size image To unambiguously link the activity of the PI compounds to the ability to metabolize glycerol, we constructed an M. tuberculosis knockout strain deficient for the expression of GlpK (MTBΔ glpK ). The MTBΔ glpK mutant strain was found resistant to the PI compounds, whereas sensitivity was restored on re-introduction of a wild-type copy of glpK in the KO strain ( Fig. 2c–e ). These results showed that glycerol dissimilation is required for the anti-tubercular activity of the PI compounds. Glycerol has long been known to be the preferred source of energy and carbon for M. tuberculosis under in vitro conditions [19] , [20] , [21] , [24] , [25] . As such, glycerol is present in most standard M. tuberculosis growth media [19] , [21] , [26] , including the culture medium used here to identify the PI compounds [26] ; a bias towards glycerol-dependent killing mechanisms may thus have resulted in the selection of the PI compounds. This hypothesis was supported by the observation that PI compounds were inactive against M. tuberculosis in the absence of glycerol in the culture medium, whereas the inhibitory effects of reference compounds such as isoniazid, streptomycin and moxifloxacin were comparable ( Fig. 2f ). Similar results were obtained when using newly isolated clinical isolates of M. tuberculosis ( Supplementary Table S2 ), ruling out the possibility that the glycerol-dependent killing mechanisms of the PI compounds are restricted to the laboratory strain H37Rv, which has been propagated in vitro on glycerol-containing medium for about 100 years [27] . Finally, the absence of growth inhibitory activity of PI compounds in vivo suggests that glycerol is not a carbon source either readily available or primarily used by M. tuberculosis in mouse lungs. Accordingly, the MTB Δ glpK mutant strain colonized mouse lungs as effectively as its parental counterpart ( Fig. 3 ), showing that M. tuberculosis glycerol dissimilation is dispensable in the mouse model of tuberculosis. 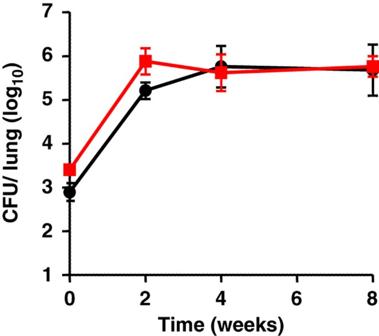Figure 3: Glycerol metabolism is not required for the virulence ofM. tuberculosis in vivo. Balb/C mice were infected intranasally with∼103bacilli of the parental H37Rv (black circles) or of the ΔglpK(red squares)M. tuberculosisstrains. The bacterial burden was followed in the lungs by CFU enumeration. Four mice per time point of each group were used and the standard deviations are shown. Figure 3: Glycerol metabolism is not required for the virulence of M. tuberculosis in vivo . Balb/C mice were infected intranasally with ∼ 10 3 bacilli of the parental H37Rv (black circles) or of the Δ glpK (red squares) M. tuberculosis strains. The bacterial burden was followed in the lungs by CFU enumeration. Four mice per time point of each group were used and the standard deviations are shown. Full size image Accumulation of glycerol phosphate in PI-treated mycobacteria The PI compounds are only active in the presence of glycerol, suggesting that they might exert their inhibitory effect by dysregulating the glycerol dissimilation pathway. Glycerol phosphate and dihydroxyacetone phosphate (DHAP) are the first two specific metabolites of the glycerol dissimilation pathway ( Fig. 5 ). As the accumulation of sugar phosphates is known to be highly toxic for most bacteria [28] , [29] , [30] , [31] , the toxicity of both metabolites was tested against M. tuberculosis . Glycerol phosphate and DHAP were added exogenously to M. tuberculosis cultures and the effect on growth was determined. Results showed that glycerol phosphate and DHAP were toxic for M. tuberculosis , showing an MIC 50 value of 12.5 and 1.2 mM respectively ( Fig. 4a ). The low potency might be because of a limited uptake of phosphorylated metabolites inside M. tuberculosis . Similarly, aldehyde methylglyoxal, a spontaneous glycolytic by-product that accumulates when the pool of sugar phosphate increases [32] , [33] , [34] ( Fig. 5 ), was also shown to be toxic, with an MIC 50 value of 0.4 mM ( Fig. 4a ). We then tested whether the PI compounds induced the intracellular accumulation of these toxic metabolites. The effect of 1 on the mycobacterial metabolome was studied by liquid chromatography/mass-spectrometry (LC/MS) 24 h after treatment. An early time point was chosen to discriminate specific changes induced by the compounds rather than by a general stress response associated with growth arrest and/or cell death. A significant accumulation of glycerol phosphate was observed specifically in cells treated with 1 and 2 ( Fig. 4b ). No changes in the levels of DHAP, or of the downstream glycolytic metabolites glyceraldehyde phosphate and pyruvate, were detected ( Fig. 4c ). These data suggested that the accumulation of glycerol phosphate might be one of the toxic consequences induced by the PI compounds in the presence of glycerol in the broth medium and of a functional glycerol dissimilation pathway. A second feature of PI compounds was the promotion of a very rapid ATP depletion in M. tuberculosis , which was not observed with the reference compounds streptomycin and moxifloxacin ( Fig. 4d ). We showed that the ATP pool was depleted by >75% in cells treated with 1 and 2 in the presence of glycerol as early as 24 h after treatment ( Fig. 4d ). Taken together, these results suggest that high intracellular levels of glycerol phosphate combined with rapid depletion of the intracellular ATP pool are specifically associated with the anti-tubercular activity of the PI compounds. Figure 5: Glycerol metabolites and the putative methylglyoxal-detoxification pathway in M. tuberculosis . 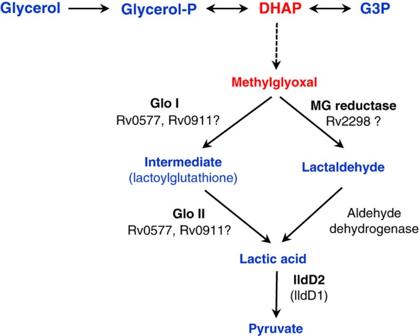Figure 5: Glycerol metabolites and the putative methylglyoxal-detoxification pathway inM. tuberculosis. The generation of methylglyoxal from DHAP is usually spontaneous (dotted line). Glo I: glyoxylase I, Glo II: glyoxylase II, lldD: lactate dehydrogenase (cytochrome), G3P: glyceraldehyde-3-phosphate, DHAP: dihydroxyacetone phosphate. The generation of methylglyoxal from DHAP is usually spontaneous (dotted line). 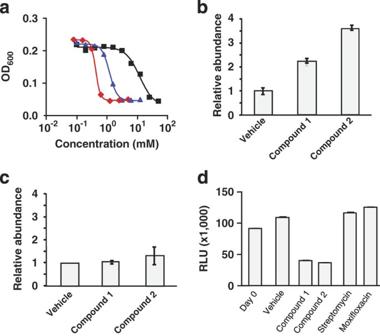Glo I: glyoxylase I, Glo II: glyoxylase II, lldD: lactate dehydrogenase (cytochrome), G3P: glyceraldehyde-3-phosphate, DHAP: dihydroxyacetone phosphate. Figure 4: Accumulation of glycerol phosphate and rapid ATP depletion in PI-treatedM.tuberculosis. (a) MIC50values of glycerol phosphate (black squares), DHAP (blue triangles) and methylglyoxal (red diamonds) were determined forM. tuberculosisH37Rv.M. tuberculosisH37Rv was exposed to1and2in the presence of glycerol for 24 h. The relative abundances of glycerol phosphate (b) and of pyruvate (c) are shown.M. tuberculosisH37Rv was exposed to1and2in the presence of glycerol for 24 h. The intracellular ATP level was quantified (d). Streptomycin and moxifloxacin were used as reference compounds. Full size image Figure 4: Accumulation of glycerol phosphate and rapid ATP depletion in PI-treated M. tuberculosis. ( a ) MIC 50 values of glycerol phosphate (black squares), DHAP (blue triangles) and methylglyoxal (red diamonds) were determined for M. tuberculosis H37Rv. M. tuberculosis H37Rv was exposed to 1 and 2 in the presence of glycerol for 24 h. The relative abundances of glycerol phosphate ( b ) and of pyruvate ( c ) are shown. M. tuberculosis H37Rv was exposed to 1 and 2 in the presence of glycerol for 24 h. The intracellular ATP level was quantified ( d ). Streptomycin and moxifloxacin were used as reference compounds. Full size image The effects triggered by the PI compounds, that is, accumulation of glycerol phosphate combined with rapid ATP depletion, reproduce almost entirely the phenotypes described for an Escherichia coli glycerol phosphate dehydrogenase knockout mutant [35] , suggesting that glycerol phosphate dehydrogenase may be the primary target of the PIs. However, we developed an enzymatic assay from M. tuberculosis cell-free extracts and showed that PI compounds do not directly inhibit M. tuberculosis glycerol phosphate dehydrogenase activity (data not shown). Putative glyoxylase rv0577 is a candidate target of PIs To identify the candidate targets of the PI compounds, an affinity chromatography approach was undertaken, whereby an active PI derivative (compound 4 , Fig. 1 ) covalently linked to sepharose beads was co-incubated with mycobacterial cell lysate, in both the presence and the absence of unbound 4 . Bound proteins were separated in parallel by SDS–polyacrylamide gel electrophoresis, trypsin-digested and identified by mass spectrometry. A quantitative comparison of these experiments identified four candidate proteins (Rv0577, Rv0911, Rv2298 and lldD2) predicted to be involved in the methylglyoxal detoxification pathway ( Fig. 5 ), the binding of which dramatically decreased in the presence of free 4 . Specifically, Rv0577, Rv2298 and Rv0911 are homologues of known glyoxylases or aldo/keto reductases, whereas lldD2 is annotated as a non-respiratory lactate dehydrogenase (cytochrome). The most abundant of the four proteins, Rv0577, was chosen for further investigation as a potential target of the PI compounds, and thus an M. tuberculosis strain overproducing Rv0577 (MTB pMV262- rv0577 ) was constructed. Interestingly, MTB pMV262- rv0577 multiplied 25% faster than the parental strain on glycerol-containing medium. This observation suggests that the product of rv0577 might participate in the detoxification of glycerol metabolism by-products. It is important to note that MTB pMV262- rv0577 showed an increased resistance to 1 and 2 compared with the parental strain ( Table 3 ), strongly supporting the notion that Rv0577 is one of the primary targets of the PI compounds. Table 3 Overexpression of Rv0577 confers resistance to PI compounds in M. tuberculosis . Full size table Historically, the discovery of new antibiotics has been primarily serendipitous. Although the value of this approach is unquestionable, little has been learned from the successes and failures encountered in the processes. Current antibiotics are mainly derived from natural sources and inhibit conserved macromolecular machineries such as DNA replication, protein or cell-wall synthesis. This narrow set of targets is truly and intrinsically essential for cell multiplication independent of the environment. With the explosion of drug resistance, there is a need to move from these historical targets to new and less conventional ones. However, the validation of new targets is more complex, as their essentiality might well be conditional and/or contextual. For instance, the metabolic target isocitrate lyase (ICL) of M. tuberculosis is strictly essential in vivo , yet dispensable under classical in vitro culture conditions [36] , [37] . In this work, we report on the underappreciated importance of the culture medium composition, and in particular the nature of the carbon source, for anti-tuberculosis drug discovery. A new class of PI inhibitors was identified from a chemical genetic screen. The PI compounds were potent in glycerol-containing medium in vitro , but without in vivo efficacy. These compounds were shown to be inactive against M. tuberculosis in the absence of glycerol or of a functional glycerol dissimilation pathway. Treatment with PI compounds resulted in the accumulation of glycerol phosphate coupled with rapid and sustained ATP depletion, thereby impairing M. tuberculosis growth and survival. Accumulation of sugar phosphate is known to be toxic for most prokaryotic and eukaryotic cells, but the basis of such toxicity is yet to be fully understood [28] , [29] , [30] , [31] , [35] . In E. coli , unregulated glycerol metabolism triggers the spontaneous formation of toxic aldehyde methylglyoxal, the latter reacting with DNA and proteins, thus promoting the accumulation of advanced-glycated end products and cell death [38] . Methylglyoxal is highly unstable and hence could not be detected in PI-treated mycobacteria. Nevertheless, affinity chromatography experiments identified four putative enzymes involved in methylglyoxal detoxification as a potential target for the PI compounds. The most abundant protein identified by affinity chromatography was Rv0577. Strikingly, overproduction of this putative glyoxylase in M. tuberculosis resulted in a strong resistant phenotype to PI compounds, conceivably establishing a link between the antimycobacterial activity of the PI compounds and methylglyoxal detoxification in the bacterium. The mechanism by which methylglyoxal is eliminated has not been studied in M. tuberculosis . Methylglyoxal is usually converted into pyruvate by lactate ( Fig. 5 ). Glutathione has a central role in methylglyoxal detoxification in enterobacteria and human cells, functioning as a cofactor for most glyoxylases. M. tuberculosis does not produce glutathione and must therefore use an alternate cofactor that remains to be identified. Further validation is required to understand the precise molecular mode of action of the PI compounds, and the link between the methylglyoxal detoxification pathway, the accumulation of toxic levels of glycerol phosphate and the depletion of the intracellular ATP pool. Two additional potent compound series from the hit list were also found to be glycerol dependent, arguing for a bias in the screening process. Such bias may be explained by the design of the screen itself; mycobacteria were exposed to the compounds for only 48 h (two-generation times) and ATP was used as an indicator of cell biomass increase. Treatment with PI compounds triggered ATP depletion as early as 24 h after incubation, a timeframe in which known antibiotics have no effect, thus favouring the selection of those inhibitors the mode of action of which involves rapid ATP depletion. Such fast-acting properties are shared by compounds that target the glycerol dissimilation pathway, explaining the observed bias towards the selection of glycerol-dependent inhibitors. Several mechanisms might explain the rapid ATP depletion observed on treatment with PI compounds. The uncontrolled phosphorylation of glycerol may function as an ATP sink, depleting the available ATP pool as described in E. coli [35] . Alternatively, glycerol phosphate may lower ATP content through a direct inhibition of oxidative phosphorylation, as recently described for maltose phosphate in M. tuberculosis [39] . Complex host-derived lipids have been proposed to represent an essential source of carbon and energy for M. tuberculosis in vivo , as evidenced by the attenuated phenotype of an M. tuberculosis strain deficient for ICL activity [19] , [21] , [25] , [36] , [37] . However, M. tuberculosis ICL is an enzyme with dual functions involved in two distinct pathways [40] , and the glyoxylate shunt is required for growth not only on lipids but also on branched-chain amino acids, alcohol and sterols. It thus remains to be determined which carbon source(s) are used by M. tuberculosis in host tissues. Finally, it is important to note that the results of studies on the mechanism of action of the PIs reported here have implications for how we approach antibacterial drug discovery. The current concept is to inhibit an essential bacterial function, assuming that this would result in growth inhibition and death of the bacterium. However, the PIs show us a possible alternative approach, derailing metabolic subsystems resulting in accumulation of toxic metabolites (for example, sugar phosphates) and the collapse of core homeostatic systems (for example, ATP level maintenance). The conceptual similarities to other recent works showing how bactericidal antibiotics truly function are striking [13] , [14] . Specifically, bacterial cell death is caused not by simple target inhibition but by complex events that occur after primary target modulation [13] , [14] . Therefore, targeting metabolic pathways known to generate toxic intermediates, such as the methylisocitrate cycle [41] , [42] , [43] , could represent an interesting approach to finding new antibacterials. In the light of the findings reported here, we believe that an in-depth knowledge and understanding of central bacterial metabolism within host tissues is required for the rational discovery of new drugs effective against M. tuberculosis and other pathogenic bacteria. Strains and growth conditions M. tuberculosis H37Rv (ATCC, cat. no. 27294) and derivative strains were maintained in Middlebrook 7H9 broth medium supplemented with 0.2% glycerol, 0.05% Tween 80 and 10% ADS supplement. Alternatively, 7H9 medium without glycerol or Sauton medium [21] was used. Culture media were supplemented with hygromycin (50 μg ml −1 ) or kanamycin (20 μg ml −1 ) when required. High-throughput cell-based screen M. bovis BCG was cultured to an OD 600 of 0.5–0.6 in complete 7H9 broth medium. In preparation for 1536-well dispensing, the culture was diluted to an OD 600 of 0.01 using complete 7H9 media. A volume of 4 μl of complete 7H9 media was dispensed into a white, solid bottom 1536-well plate using a custom Bottle Valve liquid dispenser (GNF). A volume of 100 nl of test compound in DMSO (1 mM) was then transferred into each assay plates using a custom 1536 Pintool (GNF). Diluted culture (4 μl) was subsequently added to the assay plates using a Bottle Valve liquid dispenser (final OD 600 in 8 μl is 0.005). The plates were incubated at 37 °C for 48 h. Growth was assessed by measuring ATP levels using the BacTiter-Glo Microbial Cell Viability Assay (Promega). Luminescence was measured using a ViewLux plate reader. MIC 50 determination MIC 50 were determined as previously described, with slight modifications [44] . Briefly, compounds dissolved in 90% DMSO were twofold serial-diluted in duplicates and spotted by mosquito HTS (TTP LabTech) to 384-well clear plates, resulting in 10 dilutions of each compound. A volume of 50 μl of M. tuberculosis culture (final OD 600 of 0.02) was added to each well, and the assay plates were incubated at 37 °C for 5 days. OD 600 values were recorded using a SpectraMax M2 spectrophotometer, and MIC 50 curves were plotted using GraphPad Prism 5 software. Under the assay setting, MIC 50 values, which fall in the linear part of the inhibition curve, are more robust and reproducible than MIC 90 . Therefore, only MIC 50 values are reported. Cytotoxicity Cytotoxicity was tested against cell lines HepG2 (ATCC, cat. no. HB-8065) and BHK21 (ATCC, cat. no. CCL-10) in 96-well microplates. The cells were seeded at a density of 10 5 cells per well, incubated at 37 °C for 24 h and exposed to twofold serial-diluted compounds for 3 days. Cell viability was monitored using the Cell Proliferation Kit II (Invitrogen). Selection of spontaneous PI-resistant mutants M. tuberculosis H37Rv was spread onto 7H11 plates containing 20 μM of the test compounds. Colonies were picked after 3 weeks of incubation at 37 °C and propagated into 7H9 medium. The resistance phenotype to the PI compounds was confirmed by testing MIC 50 values against 1 and 2 . Full-genome sequencing Whole-genome fragment libraries were prepared using Paired-End Sample Preparation Kit (Illumina). Briefly, 5 μg of each genomic DNA sample was fragmented using the nebulization technique for 10 min with compressed air of 32 p.s.i. The ends were repaired with the addition of A base on the 3′ end and by ligation of paired-end adaptor oligo mix. Samples were then gel-purified and selected for 200 bp fragment size to be amplified by PCR, followed by gel purification. DNA samples were hybridized onto the flowcell using a Paired-End Cluster Generation Kit v1, transferred to the Genome Analyzer Classic and 48 cycles of sequencing were performed using the 36 Cycle Sequencing Kit v2. Data Collection Sequence Control software version 2.3 was used on the Genome Analyzer I, and Pipeline version 0.3.0 was used for analysis. The resulting 7.8–9.6 million reads were aligned to the M. tuberculosis H37Rv sequence using SOAP software. Nucleotide changes from the reference sequence were called in situations in which at least six separate reads called the alternate letter, and in which the sum of the Solexa quality scores for the alternate letter was fivefold greater than the sum of the Solexa quality score for the reference letter. Insertions and deletions were verified by assembling de novo contigs with Velvet. Construction of the MTBΔ glpk strain The glpk gene was knocked out by allelic exchange using plasmid pYUB854 [45] as previously described [4] . The mutant strain MTBΔ glpk was complemented with a wild-type copy of the glpK gene under the control of its own promoter and cloned into vector pMV306 [46] . Pharmacokinetic properties and oral bioavailability CD-1 female mice were used for PK studies. The compounds were formulated in 27% HPβCD, 6-N HCl, 27% PBS and 27% citrate buffer (pH 4). The lung distribution properties of compounds were determined by LC/MS after a single dose of 25 or 100 mg kg −1 of body weight. Mouse efficacy studies In vivo efficacy studies were determined after intranasal infection of BALB/c mice with 10 3 M. tuberculosis H37Rv. Treatment was initiated 1 week after infection. Compounds were administered daily by gavage for 28 consecutive days. Bacterial loads were determined at 14 and 28 days after the initiation of treatment. All procedures involving mice were reviewed and approved by the institutional animal care and use committee of the Novartis Institute for Tropical Diseases. Metabolomics For metabolomic profiling studies, M. tuberculosis was cultivated on modified 7H10 agar plates. Bacteria were metabolically quenched by rapid transfer of bacteria-laden filters into acetonitrile/methanol/H 2 O (40:40:20), precooled to −40 °C, and metabolites were extracted by mechanical lysis, followed by clarification and filtration across a 0.22 μm filter. Bacterial biomass of individual samples was determined by measuring the residual protein content. Metabolites were separated and analysed by dual-mode electrospray ionization time-of-flight mass spectrometry using an Agilent Accurate Mass 6220 TOF. Dynamic mass axis calibration was achieved by continuous infusion of a reference mass solution using an isocratic pump with a 100:1 splitter. This configuration achieved mass errors of approximately five parts per million, mass resolution ranging from 10,000 to 25,000 (over m / z 121–955 amu) and a 5 log 10 dynamic range. Detected ions were deemed metabolites on the basis of unique accurate mass-retention time (AMRT) identifiers for masses showing the expected distribution of accompanying isotopomers. Metabolite identities were established by querying against a prepopulated AMRT library of metabolite standards and showing chromatographic co-elution of candidate metabolites with pure chemical standards spiked into representative biological samples. Determination of intracellular ATP levels The intracellular ATP level was quantified as previously described [47] . Briefly, 25 μl of M. tuberculosis culture was mixed with an equal volume of freshly prepared BacTiter-Glo reagent in white 384 flat-bottom plates and incubated in the dark for 5 min. Luminescence was measured using a Tecan Safire 2 plate reader. Protein pull-down experiments M. bovis BCG was grown to an OD 600 of 1 in 7H9 medium. Cells were disrupted by bead-beating, and protein lysates were clarified by centrifugation. 4 was coupled to NHS-sepharose beads and incubated with 5 mg of M. bovis BCG of protein lysate in the either presence (competition) or absence (control) of free 4 . After three washing steps, bound proteins were separated in parallel by SDS–polyacrylamide gel electrophoresis, trypsin-digested and identified by LC/MS. Proteins that were identified with high confidence in repeat analyses of competition pull-downs but were absent or at greatly reduced levels as indicated by spectral counting in control pull-downs were reported as potential targets. Overexpression of Rv0577 in M. tuberculosis Rv0577 was amplified by PCR and cloned into the multicopy expression vector pMV262 under the control of the mycobacterial hsp60 promoter [46] . How to cite this article: Pethe, K. et al . A chemical genetic screen in Mycobacterium tuberculosis identifies carbon-source-dependent growth inhibitors devoid of in vivo efficacy. Nat. Commun. 1:57 doi: 10.1038/ncomms1060 (2010).